High Molybdenum availability for evolution in a Mesoproterozoic lacustrine environment Trace metal data for Proterozoic marine euxinic sediments imply that the expansion of nitrogen-fixing cyanobacteria and diversification of eukaryotes were delayed while the availability of bioessential metals such as molybdenum in the ocean was limited. However, there is increasing recognition that the Mesoproterozoic evolution of nitrogen fixation and eukaryotic life may have been promoted in marginal marine and terrestrial environments, including lakes, rather than in the deep ocean. Molybdenum availability is critical to life in lakes, just as it is in the oceans. It is, therefore, important to assess molybdenum availability to the lacustrine environment in the Mesoproterozoic. Here we show that the flux of molybdenum to a Mesoproterozoic lake was 1 to 2 orders of magnitude greater than typical fluxes in the modern and ancient marine environment. Thus, there was no barrier to availability to prevent evolution in the terrestrial environment, in contrast to the nutrient-limited Mesoproterozoic oceans. The content of Molybdenum (Mo) in ancient carbonaceous shales is a valuable indicator of palaeo-redox conditions. Both the bulk concentration of Mo and the ratio of Mo to total organic carbon (% TOC) have been used to track the concentration of Mo in sea water through geologic time [1] , [2] , [3] , [4] , [5] , [6] , [7] . The data have been used particularly to infer the record of availability of nutrients in the ocean to allow the expansion of N-fixing cyanobacteria and the diversification of eukaryotic life [1] , [5] , [8] , [9] , [10] . However, growing evidence for the importance of shallow marine or terrestrial environments to the development of both N fixers and eukaryotes [11] , [12] , [13] , [14] requires an assessment of nutrient availability to the Mesoproterozoic surficial environment. Molybdenum is a key element limiting life in lakes, especially through control of N-fixation [15] , [16] , [17] , [18] . Most of the Mo supplied to the oceans is derived from weathering of the continents [6] , [19] , [20] . Lakes and other terrestrial environments are important reservoirs for the Mo between weathering and entry to the marine environment [21] , [22] . Lake sediments can exhibit significant enrichment in Mo relative to the surrounding bedrock composition [23] . For example, lake sediments in Canada and Sweden show concentrations of Mo 1 to 2 orders of magnitude greater than in parent granites [21] , [24] . Thus, ancient lake sediments are a good archive of Mo availability. Well-preserved Mesoproterozoic lacustrine sediments of 1.18 Ga age occur in the Stoer Group, Torridonian Supergroup, UK [25] . The 2-km-thick Stoer Group was deposited in an extensional setting on the passive margin of the palaeocontinent Laurentia [26] , [27] , [28] . The basin was a few hundred kilometres from the ocean, unconformable upon a basement of Lewisian (Archaean) gneisses. Provenance, palaeocurrent and sedimentological studies all indicate that the Stoer Group sediments were derived from the Lewisian basement. Rapid lateral and vertical fluctuations in coarse to fine siliciclastic facies (breccias, conglomerates, sandstones, mudrocks) and variability/reversals in palaeocurrent data are regarded as characteristically continental [26] , [28] . Almost all of the rocks are red-coloured, also characteristically continental. Depositional environments are interpreted as alluvial fans, fluviatile, aeolian and lacustrine, interfingering with each other. Laminated mudrocks are interpreted as lacustrine. Numerous horizons of desiccation cracks indicate emergence from shallow water in most lacustrine rocks. A single unit of sulphide-bearing black shale/laminated limestone is interpreted as a permanent lake deposit. Outcrop over 40 km suggests a minimum area of ∼ 1,000 km 2 for the lake basin, but possibly only 10% (100 km 2 ) may have deposits of sulphidic black shale. Clay geochemistry data confirm that this unit is lacustrine, not marine [29] . Pseudomorphs after gypsum occur in both the black shale and red beds. The climate was semi-arid, in palaeo-latitudes between 20 and 30° N (refs 30 , 31 ). The high sedimentation rate of the Stoer Group, characteristic of a continental basin, means that the carbon burial rate in lake sediments was much higher than in contemporary marine sediments [32] . A single marker horizon consisting of fine red sediment mixed with melt fragments (Stac Fada Member) is interpreted as an impact ejecta deposit [33] . Ar–Ar analysis of authigenic K-feldspar in the impact deposit yields a date of 1.18 Ga (ref. 25 ). The rocks have experienced mild metamorphism, but all sedimentary features are well preserved [26] and the sedimentary geochemistry is undisturbed [34] .The Stoer Group sediments present an unparalleled opportunity for measurement of Mo flux because the timescale of sedimentation can be measured accurately. By analogue with recent lake deposits, it has been demonstrated that the lacustrine lamination was annual [35] . This interpretation was augmented by the discovery of solar cycles within the laminated succession [35] . Therefore, the rate of deposition and the Mo concentration can be measured to yield a burial flux. The calculated Mo flux for the Stoer Group black shales is 1 to 2 orders of magnitude greater than typical Mo fluxes in the modern and ancient marine environment. Both Mo levels and Mo/TOC ratios are more comparable to values in much younger Phanerozoic marine black shales than Proterozoic marine black shales. The Mo is resident in both organic matter and sulphides, as in modern lakes. The Mesoproterozoic lacustrine environment, therefore, represented an important reservoir for Mo. The high Mo levels indicate that there was no barrier to the availability of Mo to prevent evolution in the terrestrial environment, in contrast to the nutrient-limited Mesoproterozoic oceans. Burial rates The Stoer Group includes a single unit of finely laminated, pyritic black shale within the Poll a’Mhuilt Member at Bay of Stoer ( Fig. 1 ), interpreted as the deposit of a stratified, sulphate-rich lake [26] . All samples were collected from this section (for precise locations see Supplementary Fig. 1 ), at National Grid Reference NC 032285. This unit has yielded a microfossil assemblage [26] , a record of solar cyclicity [35] and sulphur isotope data indicative of microbial activity [36] . 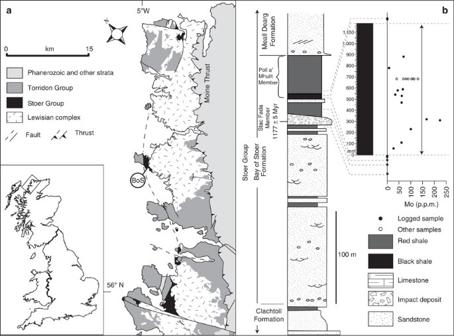Figure 1: Study area of NW Scotland and details of sample localities. (a,b) Mo values are high in black shale unit, low in other rocks. Section and regional geology adapted from ref.26. Expanded grey section represents a 1.2-m section at the base of 6 m black shale, archived in the School of Geosciences, University of Aberdeen. Logged samples are from specific levels in archived section; other samples are not located precisely within the section, but are all from within the black shale. BoS indicates Bay of Stoer sampling locality. The lamination indicates a burial rate averaging 0.27 mm per year (see Supplementary Table 1 ). This rate, in common with lacustrine sedimentation rates in general [37] , greatly exceeds rates in the deep ocean. Figure 1: Study area of NW Scotland and details of sample localities. ( a , b ) Mo values are high in black shale unit, low in other rocks. Section and regional geology adapted from ref. 26 . Expanded grey section represents a 1.2-m section at the base of 6 m black shale, archived in the School of Geosciences, University of Aberdeen. Logged samples are from specific levels in archived section; other samples are not located precisely within the section, but are all from within the black shale. BoS indicates Bay of Stoer sampling locality. Full size image Molybdenum contents Measurements of the Mo content in 20 samples of black shale and 7 samples from the overlying/underlying succession, show that there is a marked enrichment of Mo in the black shale compared with the background. The black shales have a wide range of Mo contents, with maximum and mean contents of 232 p.p.m. ( Figs 1 and 2 ) and 82 p.p.m., respectively ( Supplementary Table 1 ). The background samples average 0.7 p.p.m. The mean total organic carbon (TOC) content of the shale is 0.27%. Mo/TOC ratios are up to 859, with a mean of 304. Re/Mo ratios are in the range 10 −5 to 10 −3 ( Fig. 3 ), consistent with euxinic conditions of deposition [38] . 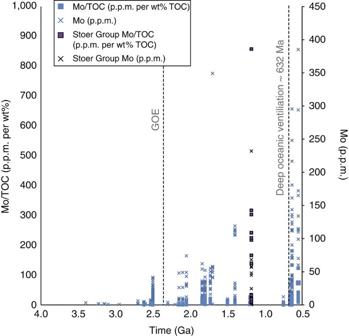Figure 2: Compilation of Mo concentrations and Mo/TOC ratios for black shales deposited under euxinic conditions. One point is shown for each sample. The mean Mo content (82 p.p.m.) for Stoer Group black shales is over three times that of Proterozoic marine shales. The mean Mo/TOC value for Stoer Group black shales (304 p.p.m. per wt%) is substantially higher than the Proterozoic average of 6.4 p.p.m. per wt%. Marine data from ref.6. GOE, great oxidation event. Figure 2: Compilation of Mo concentrations and Mo/TOC ratios for black shales deposited under euxinic conditions. One point is shown for each sample. The mean Mo content (82 p.p.m.) for Stoer Group black shales is over three times that of Proterozoic marine shales. The mean Mo/TOC value for Stoer Group black shales (304 p.p.m. per wt%) is substantially higher than the Proterozoic average of 6.4 p.p.m. per wt%. Marine data from ref. 6 . GOE, great oxidation event. 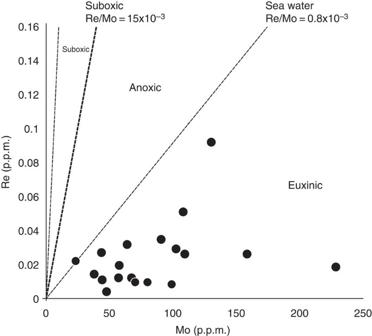Figure 3: Cross-plot of Mo and Re concentrations for Stoer Group black shale samples. Reference fields38show that Stoer Group shales were deposited in a euxinic environment. Other samples have Re contents below the detection limit. Full size image Figure 3: Cross-plot of Mo and Re concentrations for Stoer Group black shale samples. Reference fields [38] show that Stoer Group shales were deposited in a euxinic environment. Other samples have Re contents below the detection limit. Full size image Sulphur contents The Stoer Group samples have a mean sulphur content of 2.2%, and S/C ratios averaging 8.5, indicating deposition in a sulphidic setting, most commonly characteristic of marine rocks but also sulphate-rich lacustrine basins [39] . Mo is readily sequestered in sulphidic environments, where hydrogen sulphide is generated in the water column or pore waters by microbial sulphate reduction, and the Mo is partially incorporated in authigenic sulphide minerals, either directly or via thiomolybdates [1] , [3] , [18] . Accordingly, in the Stoer Group, the Mo is a trace component of pyrite, which precipitated early, before compaction of the host shale, due to microbial reduction of sulphate in the lake waters [36] . Mo in modern euxinic stratified lake waters is similarly sequestered rapidly into iron sulphides [40] , [41] . A broad correlation between Mo content and S content ( Supplementary Fig. 2 ) reflects this residence of some Mo in the Stoer Group pyrite. However, element maps show that much Mo is also resident in the organic matter-rich laminae ( Supplementary Fig. 3 ). Laser ablation-inductively coupled plasma-mass spectrometry analysis of the pyrite confirms that some Mo is resident there, at concentrations of up to 1,000 p.p.m. In addition to pyrite, the Stoer Group shale contains authigenic cadmium sulphide (greenockite), which suggests precipitation from a sulphidic water column [42] . The mean Mo content of the Stoer Group shale is over three times the average Mo content in Precambrian euxinic shales, which is ∼ 25 p.p.m. (ref. 1 ). The concentration of Mo is especially remarkable given the high sedimentation rate of the Stoer Group sediments, as other studies suggest that a high sedimentation rate dilutes the authigenic enrichment of trace metals including Mo [3] , [43] . The Mo/TOC data are much higher than the Proterozoic average of 6.4 p.p.m. per wt% (ref. 2 ). Mo/TOC ratios in marine euxinic sediments [1] , [4] , [6] remained <25 until a marked increase in atmospheric oxidation at the end of the Proterozoic. The Mo enrichments and elevated Mo/TOC ratios are more similar to those of Phanerozoic marine black shales than Proterozoic black shales ( Fig. 2 ), reflecting the high degree of sulphidation in the Stoer Group shales. The variability in the Mo/TOC results in some scatter on a cross-plot of Mo versus TOC ( Supplementary Fig. 4 ), contrary to the more coherent trends normally exhibited by these components [44] , which further indicates that the Mo content is controlled by both the S content and TOC content. Possibly the Mo was first associated with organic matter as a molybdate, as in modern anoxic lakes [45] , then partially reacted with sulphide to precipitate out. The Mo/TOC ratios are particularly high because the carbon content of the Stoer Group shales is comparatively low. The carbon content would have been higher before thermal maturation and liberation of hydrocarbons, but still probably <1% TOC. Nevertheless, at the relatively low levels of oxygenation in the Mesoproterozoic, lake stratification would have occurred readily and engendered the euxinic conditions, which precipitated sulphide minerals and sequestered trace metals including Mo. The combination of sedimentation rate and molybdenum content for individual samples allows the determination of Mo burial flux data. Sixteen samples yield a range of Mo fluxes from 2.7 to 14 × 10 −4 mol Mom −2 a −1 ( Supplementary Fig. 5 ). The mean values for burial rate and Mo content give a Mo flux of 6.5 × 10 −4 mol Mom −2 a −1 . These values are comparable with those in some modern lakes [22] , [23] , and in modern anoxic marine sediments [44] , despite much lower carbon contents ( Fig. 4 ; Supplementary Table 2 ). The values are 1 to 3 orders of magnitude higher than in modern continental margin sediments [19] ( Fig. 4 ). Comparison can be made with fluxes from episodes of anoxic marine sedimentation in the Phanerozoic geological record. Black shales from the Cambrian Alum Shale (Sweden), Ordovician Dictyonema shale (Norway), Jurassic Kimmeridge Shale (England) and Cretaceous Oceanic Anoxic Event II (USA) record fluxes 1 to 3 orders of magnitude less than in the Stoer Group (data sources in refs 19 , 22 , 23 , 44 , 46 , 47 , 48 , 49 , 50 , 51 , 52 , 53 , 54 , 55 , 56 and Supplementary Table 2 ). 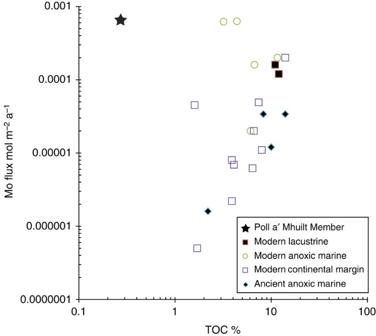Figure 4: Molybdenum burial fluxes for modern and ancient sediments. The mean flux for the Stoer Group is comparable with those in modern anoxic environments, and exceeds modern continental margins and ancient black shales. Data plotted against mean organic carbon contents (data sources in refs19,22,23,44,46,47,48,49,50,51,52,53,54,55,56andSupplementary Table 2). Figure 4: Molybdenum burial fluxes for modern and ancient sediments. The mean flux for the Stoer Group is comparable with those in modern anoxic environments, and exceeds modern continental margins and ancient black shales. Data plotted against mean organic carbon contents (data sources in refs 19 , 22 , 23 , 44 , 46 , 47 , 48 , 49 , 50 , 51 , 52 , 53 , 54 , 55 , 56 and Supplementary Table 2 ). Full size image Data from the Stoer Group indicate that Mo was being sequestered before it reached the open ocean, in this case in a euxinic lake. In lakes that were not euxinic, Mo would not be sequestered to the same degree. However, in a separate study, a more limited contrast between Mo levels in epicratonic (higher contents) and craton margin (lower contents) marine sediments of 1.1 Ga age [6] similarly suggests an ocean-ward gradient of declining Mo availability. An important control on high Mo levels in the Stoer Group was the high content of sulphide in the lake water, which reflects a high enough level of atmospheric oxygenation to allow ready weathering of sulphides on the continents [36] and hence the ready availability of sulphate to surface environments in the late Mesoproterozoic. Mo is essential to biological N fixation [57] , [58] , [59] , so the record of Mo availability to the Stoer Group lake supports models in which N-fixing cyanobacteria could flourish in the Mesoproterozoic lacustrine environment while being inhibited in the ocean. The high burial rates for Mo in the Stoer Group could be interpreted to imply a high concentration of Mo in the water column, assuming steady-state conditions. However, the Mo levels in the waters of modern lakes with Mo-rich sediments are low [22] , [23] , so the Stoer Group lake waters may not have had exceptional Mo concentrations. Nevertheless, the high Mo levels in the sediments imply that Mo input to the lake was not a limiting factor. The critical advantage to the availability of Mo in the lacustrine environment compared with the marine environment may be in the speciation of Mo, and the associated bioavailability. Mo occurs in sea water as the relatively unreactive molybdate oxyanion in the VI oxidation state, whereas in lakes up to 50% should be in the V oxidation state [16] . The anoxic conditions in a stratified lake, as envisaged for Stoer Group deposition [26] , [35] , would enhance the relative abundance of the Mo (V) form. Not only is the Mo(V) form more bioavailable [60] , [61] , but it is not inhibited by dissolved sulphate in the way that Mo (VI) is inhibited, hence the lacustrine environment strongly favours the stimulation of nitrogen fixation by its dissolved Mo content [16] . A high Mo content in the underlying lacustrine sediments may also be significant to productivity, despite low levels of Mo in lake waters, due to diffusion of Mo upwards into the water from the sediments. This additional source of Mo would allow biological uptake higher than predicted [61] . Several studies of modern lakes show that their Mo levels are adequate to support N-fixing cyanobacteria [16] , [17] , [18] , so it is possible that the Stoer Group lake was similarly adequate to host N fixers. In the particular case of a sulphate-rich lake, high availability of Mo helps to mitigate the inhibition of N fixation by the sulphate [17] . As the dating and palaeogeography of rocks of this age become better constrained [62] , it is becoming clear that sulphate deposits in continental and shallow marine deposits were more prevalent in the late Mesoproterozoic [63] than hitherto appreciated ( Supplementary Table 3 ). This implies a high potential for the sequestration of metals as sulphides, a possibility which merits further research. The Stoer Group data are also consistent with evidence for a greater diversity of eukaryotes in marginal marine environments compared with offshore marine environments, which was hypothesized to reflect the scarcity of Mo in offshore waters distant from continental run-off [13] .The availability of trace metals was a key influence on the development of multicellular life [57] , [64] , and Mo-dependent enzymes in particular are essential to eukaryotic cell biology [57] , [58] , [64] , [65] , [66] . The evolution of Mo usage is regarded as a fundamental aspect of the diversification of eukaryotes, probably from 1.5 to 1.0 Ga (ref. 58 ). The data reported here show that Mo was readily available to support such a diversification in the terrestrial environment at this critical time. Measurement of burial rates in Stoer Group samples The laminites of the Poll a’Mhuilt Member were deposited in a lacustrine setting [35] . Individual laminae comprise silt-clay, carbonate and organic components, which reflect seasonal variations in sedimentation and are comparable to annual laminae from more recent and present day lacustrine settings [35] . These annually deposited laminae allow depositional rates to be calculated with high precision from thin sections or cut and etched hand specimens. In thin section, measurement of individual laminae was possible to a precision of 10 μm using equipment originally developed for the measurement of tree rings (digital positionometer under a petrographic microscope). Depositional rates were calculated from cut and etched hand specimens by dividing the total thickness of the laminae present by the number of laminae counted under magnification. Many hundreds of laminae were measured to give high precision statistics [35] . Measurement of molybdenum contents Molybdenum and rhenium contents were measured using inductively coupled plasma-mass spectrometry (ICP-MS) using an Agilent 7,700 instrument. Samples of 100 g rock were milled and homogenized, and 0.25 g digested with perchloric, nitric, hydrofluoric and hydrochloric acids to near dryness. The residue was topped up with dilute hydrochloric acid and analysed by inductively coupled plasma-emission spectroscopy using a Varian 725 instrument. Samples with high concentrations were diluted with hydrochloric acid to make a solution of 12.5 ml, homogenized, then analysed by ICP-MS. Results were corrected for spectral inter-element interferences. The limits of detection of Mo analysis are 0.05 and 10,000 p.p.m. The lower limit of Re analysis is 0.002 p.p.m. Measurement of four standards at the same time as analysis of the Stoer Group samples fell within pre-defined target boundaries of 3–4 p.p.m., 13–17 p.p.m., 49–61 p.p.m. and 57–71 p.p.m. Analyses of blanks were <0.05 p.p.m. Mo. Duplicate analyses for blanks, standards and analysed samples were all within 1% of each other. Duplicate analyses are not plotted separately in figures. Duplicate analyses include samples processed through the entire analytical procedure. Measurement of molybdenum flux Calculations for the flux in the Stoer Group samples assume a rock density of 2.8 g cm −3 (measured on Stoer Group samples), atomic mass of molybdenum 95.94 and mean burial rate of 0.27 mm a −1 . For mean Mo content of 82 p.p.m., this equates to Mo flux of 6.5 × 10 −4 mol Mom −2 a −1 . The range of fluxes calculated is shown in Supplementary Fig. 2 . Calculations for other modern and ancient systems assume mean Mo and maximum sedimentation rates from the cited literature to give upper limits to fluxes. Where a range of TOC is cited rather than a mean value, the upper limit is used in Fig. 4 . The data plotted in Fig. 4 is shown in Supplementary Table 2 . Carbon and sulphur contents The carbon and sulphur contents of the shale were measured using a LECO CS225 elemental analyser, after decarbonatization with hydrochloric acid. Analyses are run concurrently with standards 501–024 (Leco Instruments, 3.23±0.03% C, 0.047±0.003% S, instrument uncertainty±0.05% C,±0.002% S) and BCS-CRM 362 (Bureau of Analysed Samples Ltd., 1.48% S). The repeatability of samples is consistently within 1%. Element mapping Mapping was undertaken using a Bruker M4 Tornado XRF Mapper, based at the CSIRO Advanced Characterization Facility, Perth, Australia. The mapping used a pixel size of 25 μm, with data acquired over 10 ms per pixel. The MCBM 50–0.6B Rh X-ray tube voltage was 50 kV and the anode current was 500 μA. How to cite this article : Parnell, J. et al . High Molybdenum availability for evolution in a Mesoproterozoic lacustrine environment. Nat. Commun . 6:6996 doi: 10.1038/ncomms7996 (2015).